A necessarily complex model to explain the biogeography of the amphibians and reptiles of Madagascar Pattern and process are inextricably linked in biogeographic analyses, though we can observe pattern, we must infer process. Inferences of process are often based on ad hoc comparisons using a single spatial predictor. Here, we present an alternative approach that uses mixed-spatial models to measure the predictive potential of combinations of hypotheses. Biodiversity patterns are estimated from 8,362 occurrence records from 745 species of Malagasy amphibians and reptiles. By incorporating 18 spatially explicit predictions of 12 major biogeographic hypotheses, we show that mixed models greatly improve our ability to explain the observed biodiversity patterns. We conclude that patterns are influenced by a combination of diversification processes rather than by a single predominant mechanism. A ‘one-size-fits-all’ model does not exist. By developing a novel method for examining and synthesizing spatial parameters such as species richness, endemism and community similarity, we demonstrate the potential of these analyses for understanding the diversification history of Madagascar’s biota. Interpreting the spatial distribution of biodiversity is fundamental to the study of biogeography, macroecology, evolutionary biology and conservation biology [1] , [2] . Core concepts include local and regional endemism, species richness, and species turnover, of which the two latter correspond to alpha- and beta-diversity as used in community ecology [3] , [4] . In different combinations, these core concepts are invoked to identify biogeographic regions [5] , [6] , [7] , prioritize geographic areas for conservation [8] , [9] , assess the effects of conservation measures [10] and/or delimit centres of speciation or extinction [11] . Areas of high species endemism are typically interpreted to be centres of speciation, though it is often unappreciated that these ‘areas of endemism’ are the result of numerous interacting processes that are not explicitly accounted for in the derivation of the measurement. Thus, we frequently oversimplify the dynamic and complex interactions among organisms and their environment. In practice, it is generally assumed that species formation and diversification of a range of co-distributed taxa will be either triggered or inhibited by analogous barriers to gene flow, topographical and geological settings, climatic conditions and shifts and/or competition. Accordingly, it is the default expectation that equivalent barriers (for example, rivers, ecotones, climatic transitions) will lead to congruent patterns of species endemism, turnover and richness — again, with the underlying assumption that the observation of similar patterns among diverse species reveals a general causal mechanism of diversification across all taxa. However, there are additional processes by which species richness may be generated that can act in concert with or in opposition to biogeographic barriers. For example, climatic factors, environmental stability, land area, habitat heterogeneity, palaeogeography and energy available can be spatially correlated with these barriers but not causally related to diversification [12] . Although it seems obvious that such patterns are caused by multiple mechanisms, biogeography researchers often rely on ad hoc and narrative comparisons with spatial distributions of single environmental variables such as centres of historical habitat stability [13] , climate, topography, vegetation or other assumed barriers to dispersal in searching for an assumed prevalent explanatory factor. Methodological advances are being developed to address the problems of non-uniformity and non-independence. For example, assessments of spatial biodiversity have typically used simple geographic measures as the unit of analysis, such as the distribution range of individual species, though recent methodological refinements include the integration of phylogenetic relationships among species and their evolutionary age [2] , [7] . Moreover, carefully parameterized species distribution models can generate accurate estimates of species ranges [14] and novel, more objective, approaches are being developed to translate patterns of species richness, endemism and turnover for determining those biogeographic regions in greatest need for conservation and protection [2] , [7] , [8] , [15] , [16] , [17] . Although biological explanation of these patterns is still in its methodological infancy, considerable recent development of conceptual and statistical tools now allows for integrative multivariate approaches to more realistically estimate underlying processes. Madagascar is the world’s fourth largest island and hosts an extraordinary number of endemic flora and fauna. For example, 100% of the native species of amphibians and terrestrial mammals, 92% of reptiles, 44% of birds and >90% of flowering plants occur nowhere else [18] . This megadiverse microcontinent, initially part of Gondwana, has been isolated from other continents since the Mesozoic. Its current vertebrate fauna is a mix of only a few ancient Gondwanan clades and numerous younger radiations, originating from Cenozoic overseas colonizers arriving mainly from Africa [19] , [20] , [21] . The extraordinary proportion of family-level endemism in Madagascar, and the long isolation from non-Malagasy sister lineages, provide a unique opportunity to study the mechanisms driving divergence and diversification in situ [22] . Over the past decade, numerous mechanisms and models have been formulated to explain biodiversity distribution patterns and species diversification in Madagascar, pertaining to environmental stability (or instability), solar energy input, geographic vicariance triggered by topographic or habitat complexity, intrinsic traits of organisms or stochastic effects [23] , [24] , [25] , [26] , [27] , [28] , [29] , [30] , [31] . Evidence has supported numerous hypotheses, though this evidence has typically been marshalled from limited taxa or groups of taxa with restricted phylogenetic diversity. Moreover, comprehensive statistical approaches comparing their relative importance are rare [32] . In this paper, we seek to identify the causal mechanisms that determined the spatial distribution of Madagascar’s herpetofauna by employing recent techniques that explicitly incorporate improved statistical rigour. We apply an integrative approach to simultaneously test which of the several competing and complementary hypotheses are most strongly correlated with empirical biodiversity patterns ( Fig. 1 ). We first translate a total of 12 diversification mechanisms or diversity models into explicit spatial representations. We then use univariate regressions and multivariate conditional autoregression models to assess spatial concordance of these predictor variables with species richness, endemism and turnover as calculated from original occurrence data of Madagascar’s amphibians and reptiles. Our results best agree with the hypothesis that various assemblages of species are under the influence of differing causal mechanisms, and that the distribution of diverse organismal lineages will depend on idiosyncratic factors determined by their specific organismal life-histories combined with stochastic historical factors. Thus, any model that endeavors to explain island-wide patterns must necessarily be complex. 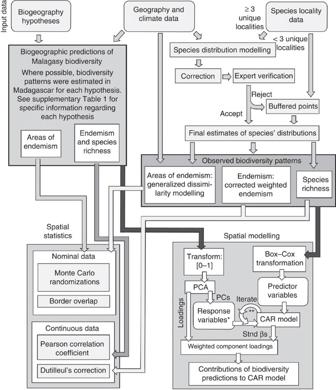Figure 1: Overview of work protocol and dataflow. Three types of original data were input into the analyses: (1) biogeography hypotheses, (2) geography and climate data and (3) species locality data. These data were used to predict the distributions of species, and the distribution models were used to calculate biodiversity patterns (species richness, corrected weighted endemism and turnover). We then tested for the correlation of these biodiversity patterns with spatial predictions derived from biogeography hypotheses, and used a mixed model to simultaneously test the influences of these hypotheses on the biodiversity patterns. *The response variables constituted standardized PCs of the raw biogeography hypotheses. ** The CAR models were iterated until only response variables that contributed significantly to the model were included. Then, the remaining variables were backward eliminated, starting with variables with smallestβs, until the AICc of the reduced model exceeded the more complex model. Figure 1: Overview of work protocol and dataflow. Three types of original data were input into the analyses: (1) biogeography hypotheses, (2) geography and climate data and (3) species locality data. These data were used to predict the distributions of species, and the distribution models were used to calculate biodiversity patterns (species richness, corrected weighted endemism and turnover). We then tested for the correlation of these biodiversity patterns with spatial predictions derived from biogeography hypotheses, and used a mixed model to simultaneously test the influences of these hypotheses on the biodiversity patterns. *The response variables constituted standardized PCs of the raw biogeography hypotheses. ** The CAR models were iterated until only response variables that contributed significantly to the model were included. Then, the remaining variables were backward eliminated, starting with variables with smallest β s, until the AICc of the reduced model exceeded the more complex model. Full size image Range sizes Mean range size (±s.d.) in our data set is smaller in amphibians than reptiles taking into account all species (41,673±55,413 km 2 versus 50,205±84,078 km 2 ; unequal variance t -test, n =679, df=649.7, t =3.981, P <0.001) and after excluding species known from only one or two localities (64,106±57,532 km 2 versus 95,294±87,495 km 2 ; unequal variance t -test, n =453, df=427.4, t =4.511, P <0.001). Microendemics (species with distributions less than 1,000 km 2 ) constitute 36.5% of all amphibian and 33.6% of all reptile species in Madagascar (difference not significant; binomial test, n =226, z =0.411, P =0.682). Spatial biodiversity patterns Species richness is highest in the eastern rainforest for both groups ( Fig. 2a,e ); in reptiles, species richness is more evenly distributed across the rainforest biome, with the area of high richness extending further into the north, west and southwest. Spatial patterns of endemism in both groups ( Fig. 2b,f ) reveal two centres of endemism, in the north around the Tsaratanana Massif and in the central east. Endemism values for reptiles are also high in southwestern Madagascar, the most arid region of the island. 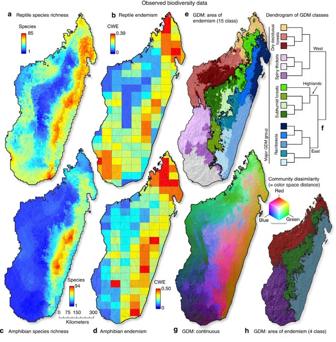Figure 2: Observed biodiversity data. Reptile species richness (a) and endemism (b). Amphibian species richness (c) and endemism (d). Species richness measures the number of species present. Endemism standardized by the local species richness and reflects the proportion of unique species present within certain areas. The GDM analyzes compositional turnover of communities (here jointly for amphibians and reptiles) and predicts dissimilarity throughout the landscape based on an interpolation of variation in climate and geographic data. (e) The 15-class GDM depicts major and minor areas of endemism. (f) The dendrogram depicts the relationships of each of the 15 classes, where sister groups comprise communities of the highest similarity. (g) The classified GDMs were generated from the continuous GDM (preclassification). This map depicts a continuous landscape where community similarity is analogous to colour space distance and the more similar colours characterize similar communities. (h) The 4-class GDM depicting major areas of endemism based on a hierarchical classification. Figure 2: Observed biodiversity data. Reptile species richness ( a ) and endemism ( b ). Amphibian species richness ( c ) and endemism ( d ). Species richness measures the number of species present. Endemism standardized by the local species richness and reflects the proportion of unique species present within certain areas. The GDM analyzes compositional turnover of communities (here jointly for amphibians and reptiles) and predicts dissimilarity throughout the landscape based on an interpolation of variation in climate and geographic data. ( e ) The 15-class GDM depicts major and minor areas of endemism. ( f ) The dendrogram depicts the relationships of each of the 15 classes, where sister groups comprise communities of the highest similarity. ( g ) The classified GDMs were generated from the continuous GDM (preclassification). This map depicts a continuous landscape where community similarity is analogous to colour space distance and the more similar colours characterize similar communities. ( h ) The 4-class GDM depicting major areas of endemism based on a hierarchical classification. Full size image We applied Generalized Dissimilarity Modelling (GDM) [33] , [34] to identify areas of endemism on the basis of turnover patterns for reptiles and amphibians together. The GDM model captured 64.4% of deviance explained. The top climatic predictors of species turnover (and percent of contribution to model) were: maximum temperature of warmest month (21.3%), precipitation of warmest quarter (19.1%), temperature seasonality (17.5%) and precipitation of driest month (12.0%). Given that the deviance explained is similar to other robust GDMs [35] , but not near 100%, non-climatic species-specific idiosyncrasies were retained in input data and support the use of the methods here. The major areas of endemism obtained in a 4-class categorization of the originally continuous GDM results ( Fig. 2h,g ) largely mirrors the bioclimatic regions of Cornet [36] . Biogeography hypotheses Our test includes a total of 12 predictor hypotheses, some of which focus on the geographical pattern in which species diversity is distributed, but without making any clear assumption about how the species originated (for example, the Mid-domain or Topographic Heterogeneity hypotheses). Others explicitly refer to mechanisms of diversification and make predictions about how these processes affected the distribution of species diversity over geographical space [36] (see Supplementary Methods and Supplementary Table 1 for detailed accounts). We divided the hypotheses into two categories: one for which continuous two-dimensional spatial richness and endemism can be derived, and the other for which only nominal areas of endemism predictions can be derived. The first category includes: Climatic Stability, Climate Gradient, Disturbance Vicariance, the Mid-domain Effect, Montane Species Pump, Museum, Refuge, Sanctuary and Topographic Heterogeneity. The second category includes climate gradient (also depicted as a continuous hypothesis), Riverine Barrier (minor and major rivers), River-Refuge and Watershed. All these hypotheses were transformed into explicit spatial representations ( Supplementary Note 1 , Supplemental Data 1 and 2 ) and used as predictor variables for further analyses. Spatial statistics We calculated unbiased correlation of the continuous predictor and test variables following the method of Dutilleul [37] , which reduces the degrees of freedom according to the level of spatial autocorrelation between two variables ( Supplementary Table 2 ). Measures of reptile and amphibian endemism were both significantly correlated with the Topographic Heterogeneity and Museum hypotheses. Amphibian endemism was also uniquely correlated to the Montane Species Pump, Disturbance Vicariance and Sanctuary hypotheses ( Supplementary Table 2 ). Correlations with species richness were not tied to measures of endemism. Whereas reptile and amphibian species richness both correlate with the Sanctuary and Museum hypotheses, the reptiles uniquely correlate with the Mid-domain Effect (distance), and amphibians uniquely with the Topographic Heterogeneity, Montane Species Pump, Disturbance Vicariance and River-Refuge hypotheses. In the univariate correlation analyses ( Table 1 ), we compared the biogeographic zonation of Madagascar as suggested by the GDM analysis of amphibian and reptile distributions ( Fig. 2c,h ) with nominal zonations derived from five predictor hypotheses ( Supplementary Fig. 1 ). We found the predictor variables corresponding to the two Riverine hypotheses and the Gradient hypothesis to be significantly correlated with both the 15- and 4-class GDMs. In addition, the River-Refuge hypothesis was significantly correlated with the 15-class GDM. Only the Watershed hypothesis was not correlated with either classification of the GDM. Both GDM classifications share the most overlap with the Gradient and the two Riverine hypotheses (25.8 – 28.8%, and 47.7 – 55.6%, for the 4- and 15-class GDMs, respectively; Table 1 ). Table 1 Correlations of nominal biodiversity hypotheses to GDMs. Full size table Mixed spatial models of biodiversity patterns Given the significant correlation of each of the spatial amphibian and reptile biodiversity patterns with various predictor variables, we used mixed conditional autoregressive spatial models (CAR models) to test the influences of various predictors simultaneously ( Supplementary Fig. 2 ). To avoid over-parameterization, we used AICc (corrected Akaike Information Criterion), an information-theoretical approach, to compare models with different sets of predictors. We found that complex models including most of the biogeography hypotheses (that were representable as continuous predictor variables) performed best, based on the lowest AICc values and consequently used these for further analysis. 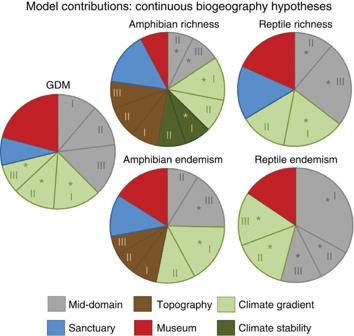Figure 3: Explanatory contribution of continuous biogeography hypotheses to a CAR spatial model of each observed biodiversity measurements. Only hypotheses contributing ≥5% are shown. Pie charts correspond to contribution of response variables in each biodiversity model (starting at left, clockwise): species turnover, amphibian species richness, reptile species richness, reptile endemism and amphibian endemism. The included response variables are numbered within each coloured group as follows: Mid-domain: I. latitude, II. longitude, III. distance. Climate gradient: I. PC1, II. PC2, III. PC3. Climate stability: I. Precipitation stability, II. Climate stability (temperature and precipitation). Topography: I. Topographic Heterogeneity, II. Disturbance Vicariance, III. Montane Species Pump. An asterisk marks hypotheses that contributed negatively to the mixed Orthogonally Transformed Beta Coefficient/CAR model. For all hypotheses (except for the climate-gradient variables), a positive correlation was expected between biodiversity metrics. Detailed contributions of each predictor to the models of species richness, endemism and GDM zonation are summarized in Supplementary Table 3 . The top-five variables contributed 49.4–75.9% to the models ( Supplementary Table 3 ). For a more simplified graphical representation ( Fig. 3 ), we summarized the three Mid-domain Effect hypotheses (latitude, longitude and distance), the three principal components (PCs) representing the Gradient hypothesis, and three hypotheses focused on topography (Topographic Heterogeneity, Disturbance Vicariance, Montane Species Pump), respectively ( Figs 3 and 4 ). We found relevant influences of the Mid-domain Effect especially on the GDM, and on the species richness and endemism of reptiles (30.9, 32.9 and 45.5%, respectively). However, it is important to point out that almost all the Mid-domain correlation coefficients were negative. Thus, indicating that factors determining spatial patterning were those inversely correlated with latitudinal and longitudinal Mid-domain Effects, that is, favouring endemism and richness at the edges rather than centre of the domain. Climate Gradient effects influenced all the models of biodiversity equally, contributing roughly a quarter to each (25.1–27.7%), though in many cases the sign of the contribution varied. However, in this case, a positive correlation was not expected. The topography variables contributed positively to the richness and endemism models of amphibians and reptiles, with joint influences of 9.1 and 22.4% on richness, and 6.5 and 17.3% on endemism. The Sanctuary and Museum hypotheses each contributed positively to all models, with Museum contributing between 7.1 and 17.1% (one of the few hypothesis to contribute >5% and to be positively correlated to all biodiversity measurements in the mixed models). The Sanctuary hypothesis also contributed positively to all mixed models, though to a lesser degree than the Museum hypothesis, and with a very low contribution to reptile endemism. Figure 3: Explanatory contribution of continuous biogeography hypotheses to a CAR spatial model of each observed biodiversity measurements. Only hypotheses contributing ≥5% are shown. Pie charts correspond to contribution of response variables in each biodiversity model (starting at left, clockwise): species turnover, amphibian species richness, reptile species richness, reptile endemism and amphibian endemism. The included response variables are numbered within each coloured group as follows: Mid-domain: I. latitude, II. longitude, III. distance. Climate gradient: I. PC1, II. PC2, III. PC3. Climate stability: I. Precipitation stability, II. Climate stability (temperature and precipitation). Topography: I. Topographic Heterogeneity, II. Disturbance Vicariance, III. Montane Species Pump. An asterisk marks hypotheses that contributed negatively to the mixed Orthogonally Transformed Beta Coefficient/CAR model. For all hypotheses (except for the climate-gradient variables), a positive correlation was expected between biodiversity metrics. 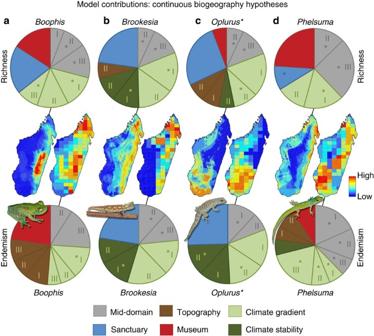Figure 4: Contribution of continuous biogeography hypotheses to a CAR spatial model of species richness and endemism for four focal groups. Only hypotheses contributing ≥5% are shown. Pie charts on top row and bottom correspond to contribution of response variables in modeling species richness and endemism, respectively. Response variables: The included response variables are numbered within each coloured group as follows: Mid-domain: I. latitude, II. longitude, III. distance. Climate Gradient: I. PC1, II. PC2, III. PC3. Climate Stability: I. Precipitation Stability, II. Climate Stability (temperature and precipitation). Topography: I. Topographic Heterogeneity, II. Disturbance Vicariance, III. Montane Species Pump. The four focal groups: (a)Brookesiachameleons (number of species=27, number of original distribution points=178), (b)Boophistreefrogs (number of species=77, number of points=460) (c)Phelsumaday geckos (number of species=28, number of points=304), and (d)Oplurusiguanas (*plus the monotypicChalarodon; number of species=7, number of points=147). An asterisk marks hypotheses that contributed negatively to the mixed Orthogonally Transformed Beta Coefficient/CAR model. For all hypotheses (with exception to the climate-gradient variables), a positive correlation was expected between biodiversity metrics. Full size image Figure 4: Contribution of continuous biogeography hypotheses to a CAR spatial model of species richness and endemism for four focal groups. Only hypotheses contributing ≥5% are shown. Pie charts on top row and bottom correspond to contribution of response variables in modeling species richness and endemism, respectively. Response variables: The included response variables are numbered within each coloured group as follows: Mid-domain: I. latitude, II. longitude, III. distance. Climate Gradient: I. PC1, II. PC2, III. PC3. Climate Stability: I. Precipitation Stability, II. Climate Stability (temperature and precipitation). Topography: I. Topographic Heterogeneity, II. Disturbance Vicariance, III. Montane Species Pump. The four focal groups: ( a ) Brookesia chameleons (number of species=27, number of original distribution points=178), ( b ) Boophis treefrogs (number of species=77, number of points=460) ( c ) Phelsuma day geckos (number of species=28, number of points=304), and ( d ) Oplurus iguanas (*plus the monotypic Chalarodon ; number of species=7, number of points=147). An asterisk marks hypotheses that contributed negatively to the mixed Orthogonally Transformed Beta Coefficient/CAR model. For all hypotheses (with exception to the climate-gradient variables), a positive correlation was expected between biodiversity metrics. Full size image To assess variation in biogeography patterns among major groups of the Malagasy herpetofauna, we calculated mixed CAR models using the same methods for richness and endemism of four exemplar sub-clades: the leaf chameleons ( Brookesia ), tree frogs ( Boophis ), day geckos ( Phelsuma ) and iguanas ( Oplurus with the monotypic iguana genus Chalarodon ). The top contributors to the models were drastically different for several of these clades ( Fig. 4 and Supplementary Table 4 ). For instance, the topography variables had strong influences on Boophis richness, with a joint contribution of 24.5%, but contributed much less to explaining the patterns of most other groups. Further, the Sanctuary hypothesis had a strong influence on the Brookesia and Oplurus models, though it contributed very little to the predictions of endemism in Boophis and Phelsuma . Mid-domain Effects were apparent in most models, but the sign of the correlation and the contribution of each Mid-domain hypothesis varied considerably. Thus, the explanatory power of this stochastic null-model is limited. We propose a novel method for examining and synthesizing spatial parameters such as species richness, endemism and community similarity. In this framework, biogeographic hypotheses are explanatory variables. The resulting mixed-model geospatial approach to biogeographic analyses is both more robust and more realistic. Our approach accounts for biological complexity in searches for prevalent factors influencing the distribution of biodiversity, both in Madagascar and elsewhere. It considerably extends univariate and sometimes narrative approaches that examine the fit of the observed patterns to only single explanatory models or mechanisms (for example, in Madagascar [27] , [29] , [38] ) or compare a limited number of competing variables in univariate approaches [32] . Such analyses might be hampered by spatial autocorrelation of biodiversity patterns and predictor variables thereby inflating type-I errors in traditional statistical tests [39] , [40] . Spatial autocorrelation can be excluded from models [41] as a predictive parameter [42] , [43] , [44] or by incorporating the spatial dependence into the covariance structure [44] , as was applied in this study. The results obtained here for some sub-clades are in agreement with previous analyses, while others are not. For example, the high influence of the Mid-domain Effect on Boophis treefrogs, one of the most species-rich frog genera in Madagascar, agrees with a previous analysis [45] for all Malagasy amphibians (with a high representation of Boophis ). On the contrary, the negative contributions of the Mid-domain Effects on the biodiversity patterns of the other genera in the analysis are not surprising given that their centres of richness and endemism are in either southern or northern Madagascar, but not in central parts of the island. Previous studies postulated a high influence of topography on the diversification of leaf chameleons ( Brookesia ) [38] , [46] , though this is not supported by our analysis. This latter example exemplifies a dilemma of scale, inherent in all comparisons of spatial data sets. In fact, the distribution of Brookesia is highly specific to certain mountain massifs in northern Madagascar, while the genus is largely absent from the equally topographically heterogeneous south-east. This absence is probably due to its evolutionary history, with a diversification mainly in the north and limited capacity for range expansion [38] . This historical distribution pattern probably accounts for low influence of the topographic hypotheses on Madagascar-wide Brookesia richness and endemism, while at a smaller spatial scale (northern Madagascar) these hypotheses might well have a strong predictive value. While patterns of richness and endemism of the Malagasy herpetofauna have been analysed several times for various purposes based on partial data sets [8] , [29] , [32] , [38] , [45] , the analysis of turnover of species composition and the definition of biogeographic regions following from such explicit analyses are still in their infancy. For reptiles, Angel’s [47] proposal of biogeographic regions based on classical phytogeography (regions based on plant community composition [48] ) has usually been adopted [49] . Later, Schatz [50] refined this zonation of Madagascar based on explicit bioclimatic analyses, and Glaw and Vences [51] proposed a detailed geographical zonation based on the areas of endemism of Wilme [27] . The GDM approach herein is the first explicit analysis of a large herpetofaunal dataset to geographically delimit regions distinguished by abrupt changes in the amphibian and reptile communities. This model turned out to agree remarkably well with classical bioclimatic and phytogeographic zonations of Madagascar [48] , [50] , and is strongly correlated to climatic explanatory variables ( Fig. 3 ). Especially in the 4-class GDM, the regions almost perfectly correspond with those proposed by Schatz [50] based on bioclimate, that is, eastern humid, central highland/montane, western arid, south-western subarid zones. Although the coincidence of the precise boundaries of these regions might be methodologically somewhat biased, as we interpolated community distribution using climate variables in the analysis, the model is still mainly based on real distributional information of species and thus provides important insights into diversification patterns of Malagasy reptiles and amphibians. Several authors have suggested that the current distribution of biotic diversity in the tropics resulted from a complex interplay of a variety of diversification mechanisms [52] , [53] . This implies that no single hypothesis adequately explains the diversification of broad taxonomic groups—our results support this assumption. Richness, endemism and turnover of large and heterogeneous groups exemplified by the all-species amphibian and reptile data sets were in all cases best explained by complex CAR models. These models have the advantage of simultaneously incorporating most or all of the originally included explanatory variables and thereby accounting for possible autocorrelation among them (as implemented here). Several alternative explanations may account for this outcome. Patterns of biodiversity may not be strongly correlated to any of the predictor mechanisms simply because none of them provide the causal mechanism underlying the diversification processes. As another consideration, spatial predictions of some of the biodiversity hypotheses may have been inaccurate, though we took great care to avoid such mistakes. In any event, improvements in these methods may result in different outcomes in future analyses. Caveats aside, the results of this study almost certainly support a third explanation that different clades of organisms are each predominantly influenced by a different set of diversification mechanisms. In turn, these are driven by intrinsic factors, such as morphological or physiological constraints, or by extrinsic factors, such as an initial diversification in an area characterized by a certain topography, climate or biotic composition. This alternative is supported by the observation that the patterns of several of the smaller subgroups in our analysis were indeed best explained by opposing predominant variables, for example, Topographic Heterogeneity and Museum ( Boophis endemism) versus Climate Stability and Sanctuary ( Brookesia endemism). An overarching message is that the taxonomic scale of analysis is of extreme importance when attempting to derive global explanations of biodiversity distribution patterns. Including too many taxa will blur the existing differences among clades and lead to complex explanatory models, whereas patterns within specific clades may be best explained by simple models. The method proposed herein allows for a more objective quantification of the influences of particular diversification mechanisms on biodiversity patterns, compared with traditional, univariate approaches. Further developments of the method should especially focus on including a phylogenetic dimension, and when appropriate (for predictor hypotheses), a temporal component. Geospatial analyses of biodiversity pattern typically use species as equivalent and independent data points, though in reality, they are entities with substantial variation in parameters such as evolutionary age, dispersal capacity and population density, and with different degrees of relatedness depending on their position in the tree of life. This multilayered information can be included in various ways in the CAR/Orthogonally Transformed Beta Coefficients approach (detailed in methods), for example, by plotting richness and endemism of evolutionary history rather than taxonomic identity, calculating turnover only for sister species with adjacent ranges or repeating the calculations for sets of species defined by particular nodes on a phylogenetic tree. This latter approach—iterating the analysis for successively more inclusive clades—appears particularly promising for identifying those moments in evolutionary history wherein shifts in prevalent diversification mechanisms have occurred. Finally, a recent spatially explicit model of geographic range evolution and cladogenesis suggests that non-constant rates of speciation can be a direct consequence of the apportioning of geographic ranges that accompanies speciation [54] . Conversely, it will be of high interest to test which kinds of spatial biodiversity patterns might arise under different speciation scenarios and their stochastic variation. Our study confirms the obvious assumption that spatial biodiversity patterns differ between major clades of organisms such as amphibians and reptiles, but also among sub-clades that evolved under different selection pressures due to their life-histories. By developing a novel method for simultaneously considering different causal processes, we can begin to tease apart the diversification histories of individual clades versus prevailing biogeoclimatic events that shape entire biotas. Accordingly, we can identify the circumstances under which life history traits versus stochastic environmental effects influence the course of evolution, and also, the settings under which selection shapes these life history traits. Species distribution modelling To understand spatial distribution patterns in Madagascar’s herpetofauna, we first compared range sizes, and computed species richness and endemism from the modelled distribution areas of amphibians and non-avian reptiles (herein called reptiles). Species data consisted of 8,362 occurrence records of 745 Malagasy amphibian and reptile species (325 and 420 species, respectively). Species distribution models were limited to species that had, at minimum, three unique occurrence points at the spatial resolution (0.91 km 2 ). The reduced dataset represented 453 species (consisting of 5,440 training points of 248 reptile and 205 amphibian species) with a mean of 12 training points per species (max=131). For 107 amphibian and 119 reptile species with only one to two occurrence records, a 10-km buffer was applied to point localities in place of modelling. The species distribution models were generated in MaxEnt v3.3.3e (ref. 55 ) using the following parameters: random test percentage=25, regularization multiplier=1, maximum number of background points=10,000, replicates=10, replicated run type=cross validate, threshold=minimum training presence. One limitation of presence-only data species distribution modelling methods is the effect of sample selection bias, where some areas in the landscape are sampled more intensively than others [56] . To optimize performance MaxEnt requires an unbiased sample. To account for sampling biases, we used a bias file representing a Gaussian kernel density of all species occurrence localities sampled at 1 decimal degree search radius [57] . The bias file up-weighted presence-only data points with fewer neighbours in the geographic landscape [58] . Species distributions were modelled for the current climate using the 19 standard bioclimatic variables (Worldclim 1.4 (ref. 59 )). Non-climatic variables (geology, aspect, elevation, solar radiation and slope) were also included [60] , [61] . All layers were projected to Africa Alber’s Equal-Area Cylindrical projection in ArcMap at a resolution of 0.91 km 2 . Correcting species distribution models for overprediction To limit geographical over-prediction of species distribution models, a problem common with modelling distributions of biota across regions with many biomes or centres of endemism [8] , [32] , we clipped each model following the approach of Kremen et al . [8] This method produces models that represent suitable habitat within an area of known occurrence (based on a buffered minimum convex polygon (MCP) of occurrence localities), excluding suitable habitat greatly outside of observed range. The size of the buffer was based on the area of the MCP. We used buffer distances of 20, 40 and 80 km, respectively, for three MCP area classes, 0–200, 200–1,000 and >1,000 km 2 . All corrected species distribution models were proofed by taxonomic experts to ensure reliability; if a model did not tightly match knowledge of areas where distributions were well documented, or if little prior information existed regarding a species distribution or taxonomy was convoluted, and because of, its expected distribution could not be evaluated, the species was excluded from analyses ( n =71). Range sizes For descriptive range-size statistics, distribution range sizes were sampled for all species at ca. 1 km 2 from corrected species distribution models (or buffered point data where applicable) and a Student’s t -test with unequal variance was performed between amphibian and reptile species. To assess differences in the frequency of microendemics among the two groups, we converted all distributions that were >or ≤1,000 km 2 to a value of 0 and 1, respectively. We then calculated the mean frequency for both groups and ran a binomial test among both groups. Species richness was calculated separately for amphibians and reptiles by summing the respective corrected binary species distribution models (based on a minimum training presence threshold) and, for species with one to two occurrence records, buffered points in ArcGIS. This provided a high-resolution estimate of richness that is less affected by spatial scale and incomplete sampling than traditional measurements based solely on occurrence records. Species richness and corrected weighted endemism Measures of endemism are inherently dependent on spatial scale. We chose a grid scale of 82 × 63 km, separating Madagascar into 24 latitudinal and eight longitudinal rows, to reduce problems associated with estimating endemism over too small or large areas [11] , [29] . Specifically, this spatial scale was chosen so that we calculated a landscape-level measure of endemism (versus fine-scale regional differences). Endemism was measured as corrected weighted endemism (CWE), where the proportion of endemics are inversely weighted by their range size (species with smaller ranges are weighted more than those with large [62] ) and this value divided by the local species richness [11] . We chose CWE over the alternative measure of (uncorrected) Weighted Endemism because it emphasizes areas that have a high proportion of animals with restricted ranges, but not necessarily high species richness, and is therefore a largely independent spatial key measure of biodiversity. We calculated CWE separately for reptiles and amphibians using SDMtoolbox v1 (ref. 57 ). GDM GDM is a statistical technique extended from matrix regressions designed to accommodate nonlinear data commonly encountered in ecological studies [33] . One use of GDM is to analyse and predict spatial patterns of turnover in community composition across large areas. In short, a GDM is fitted to available biological data (the absence or presence of species at each site and environmental and geographic data) then compositional dissimilarity is predicted at unsampled localities throughout the landscape based on environmental and geographic data in the model. The result is a matrix of predicted compositional dissimilarities (PCD) between pairs of locations throughout the focal landscape. To visualize the predicted compositional dissimilarities, multidimensional scaling was applied, reducing the data to three ordination axes and in a GIS, each axis was assigned a separate RGB colour (red, green or blue). Due to computation limitations associated with pairwise comparisons of large datasets, we could not predict composition dissimilarities among all sites in our high resolution Madagascar data set. To address this, we randomly sampled 2,500 points throughout Madagascar from a ca. 10 km 2 grid. We then measured the absence or presence of each of the 679 species at each locality. We used the same high-resolution environmental and geography data used in the species distribution model. These 23 layers were reduced to nine vectors in a PC analyses, which represented 99.4% of the variation of the original data. These data were sampled at the same 2,500 localities. Both data (species presence and environmental data) were input into a GDM using the R package: GDM R distribution pack v1.1 ( www.biomaps.net.au/gdm/GDM_R_Distribution_Pack_V1.1.zip ). We then extrapolated the GDM into the high resolution climate dataset by assigning ordination scores using k-nearest neighbour classification ( k =3, numeric Manhattan distance), calculating each ordination axes independently [33] . The continuous GDM was transformed into a model with four major classes, and each of these was then classified separately into three–five minor classes. The numbers of major and minor classes were based on hierarchical cluster analyses in SPSS v19 (ref. 63 ) using a ‘bottom up’ approach. The number of classes equaled the number of dendrogram nodes with relative distances (scaled from 0 to 1) at 0.71 and 0.63 for major and minor groups, respectively. The distance cutoff can be somewhat arbitrary; however, in our data there were obvious discontinuities (long dendrogram branches between nodes) at these two values. The resulting classified models were interpolated into high resolution climate space using a k-nearest neighbour classification as described above. Biogeography hypotheses In a GIS, spatially explicit predictions of the three biodiversity patterns (species richness, endemism and areas of endemism) [11] , [64] , [65] were estimated for each biogeography hypothesis. For some of the hypotheses, not all three metrics of biodiversity were calculated due to lacking, or incomplete, expectations (for example, not all hypotheses make predictions about areas of endemism). Because of these incomplete biodiversity pattern predictions, comparisons among hypotheses are statistically complex. This is in part because few diversification hypotheses capture all facets of biodiversity (species richness, endemism, areas of endemism). Further, many estimates of biodiversity patterns rely on components of climate or geography, thus some are based on the same data and are not entirely independent of each other. Each hypothesis was generated at the spatial resolution of 30-arc-seconds (matching the resolution of GDM and species richness estimates, later transformed to 0.91 km 2 ). For the endemism analyses, each biogeography hypothesis was upscaled to match resolution of the endemism analyses by averaging all values encompassed in each cell. Spatial statistics The spatial predictions derived from the various biodiversity hypotheses resulted in either continuous or nominal categorical data. Conducting statistical tests between data types is non-trivial and, in some cases, not logical or impossible, as these will be represented in GIS in different formats (raster and vector), and vector data furthermore can be represented by points, lines or polygons. We therefore conducted the following separate analyses to test for the influences of such different data types. Analyses of continuous data To assess a global measurement of correlation between continuous data, we calculated Pearson correlations following the unbiased correlation method of Dutilleul [37] and using the software Spatial Analysis in Macroecology [66] . Analyses of nominal categorical data Comparisons of nominal categorical spatial data (that is, areas of endemism predictions compared with the classified GDMs) focused on the spatial distributions of the borders between the subunits. Here, we asked whether turnover, as measured by our classified GDMs, occurs across similar distances with the area of endemism regions. We measured the proportion of border overlap and then the significance of this overlap using Monte Carlo spatial statistics. Madagascar was evenly sampled at 20 km 2 resulting in 1,911 sampling points. The country outline, and associated points, were excluded from all comparisons to focus analyses on the intracountry borders. The remaining 1,610 points were used in the Monte Carlo analyses of boundary overlap. To assign borders to the spatial sampling points, a 10-km buffer was applied to simplified polylines of each nominal hypothesis and all points within this buffer were classified as a border. This sampling regime applied a single point to each corresponding segment of the area of endemism boundaries. Depending on the hypothesis, the number of points depicting borders ranged from 302 to 604 units. The 4- and 15-class GDM zones were depicted by 292 and 613 points, respectively. Each hypothesis was compared with both GDM point datasets and shared borders were counted. To assess significance, Monte Carlo analyses shuffled the spatial location of the area of endemism borders among the 1610 sites ( n =10,000) and each iteration, the number of shared border points were counted. The frequency that randomized dataset exceeded the observed overlap was used to estimate the significance of the relationship between the classified GDM and each area of endemism hypothesis. Mixed models of continuous data To determine the influence of each biogeography hypothesis in predicting the observed biodiversity patterns, we integrated all continuous biogeography hypotheses into a single mixed CAR using the software Spatial Analysis in Macroecology [66] . To normalize the predictor variables, Box–Cox transformations [67] were performed. The lambda parameter was estimated by maximizing the log-likelihood profile in R package GeoR [44] . A Gabriel connection matrix was used to describe the spatial relationship among sample points [68] . Using Gabriel networks, short connections between neighbouring points, are preferable (that is, more conservative [69] ) than using inverse-decaying distances because in most empirical datasets the residual spatial autocorrelation tends to be stronger at smaller distance classes [70] . The main goal of our mixed spatial analyses were to determine the combination of biogeography hypotheses that best predict the observed biodiversity patterns. If each explanatory variable was incorporated natively, due to considerable multi-colinearity, often only a few variables would end up contributing to a majority of the model. To estimate the true contribution of each hypothesis in context of a mixed model (even if highly correlated to others), we developed a novel approach that removes colinearity from the response variables (but in the process explicit variable identity is temporarily lost). The transformed response variables are then run in a CAR analysis and the resulting standardized model contributions are then transformed back into original response variable identities; reflecting the relative contribution of each in the model. This method is herein called Orthogonally Transformed Beta Coefficients. Orthogonally transformed beta coefficients Each biogeography hypothesis was standardized from zero to one. This ensured that the component loadings reflected the relative contribution of each biogeography hypothesis. A PC analysis was performed on the standardized biogeography hypotheses using a covariance matrix. All the resulting PCs were extracted and then loaded as explanatory variables in the CAR model. The CAR analyses were run iteratively, starting with all PCs as response variables and then excluding each PC that did not contribute significantly to the model ( α =0.05) until the final model included only PCs that contributed significantly. These variables were then backward eliminated, starting with variables with smallest β coefficients, until the AICc of reduced model exceeded the more complex model. Because each PC represented a linearly uncorrelated variable, only the relevant, independent data were incorporated into the final CAR model. The resulting standardized beta coefficients ( β j from the CAR analyses, Fig. 1 and equation 1) were then multiplied by the value of the corresponding component loadings ( α ij from the PCA, see equation 1). The absolute value of the product reflects the relative contributions of each biogeography hypothesis to each PC, which are weighted by the PC’s contribution in the CAR model (herein termed the weighted component loadings or WCL if , equation 1). The weighted component loadings (WCL if , equation 1) were then summed for each biogeography hypothesis across all PCs ( H i ) and depict the contributions of each hypothesis in the CAR model. The value was then converted to percentages ( HP i ) to allow comparison among all CAR analyses. A positive or negative correlation was determined for each biogeography hypothesis by running a separate CAR analysis using the raw biogeography variables as a single response variable (all other parameters were matched). How to cite this article: Brown, J. L. et al . A necessarily complex model to explain the biogeography of the amphibians and reptiles of Madagascar. Nat. Commun. 5:5046 doi: 10.1038/ncomms6046 (2014).